Osmium evidence for synchronicity between a rise in atmospheric oxygen and Palaeoproterozoic deglaciation Early Palaeoproterozoic (2.5–2.0 billion years ago) was a critical phase in Earth's history, characterized by multiple severe glaciations and a rise in atmospheric O 2 (the Great Oxidation Event). Although glaciations occurred at the time of O 2 increase, the relationship between climatic and atmospheric transitions remains poorly understood. Here we report high concentrations of the redox-sensitive element Os with high initial 187 Os/ 188 Os values in a sandstone–siltstone interval that spans the transition from glacial diamictite to overlying carbonate in the Huronian Supergroup, Canada. Together with the results of Re, Mo and S analyses of the sediments, we suggest that immediately after the second Palaeoproterozoic glaciation, atmospheric O 2 levels became sufficiently high to deliver radiogenic continental Os to shallow-marine environments, indicating the synchronicity of an episode of increasing O 2 and deglaciation. This result supports the hypothesis that climatic recovery from the glaciations acted to accelerate the Great Oxidation Event. Earth's atmosphere is suggested to have shifted from anoxic to oxic in early Palaeoproterozoic during ~2.45–2.2 billion years ago (Ga) [1] , [2] , [3] , [4] , [5] , [6] , [7] , [8] . Any increase in O 2 would have resulted in reduced atmospheric methane levels, triggering glaciations [2] . Alternatively, dramatic geological events such as a global glaciation could have caused a shift in the balance of oxidants and reductants at Earth's surface [8] , [9] , [10] . Although several hypotheses have been proposed with regard to correlating geologic events and atmospheric transition, their relationship remains poorly constrained. To develop a more complete history of interactions in Earth's system, investigating continuous records of atmospheric O 2 levels in response to geological events is prerequisite. The abundance of redox-sensitive elements in sedimentary rocks is a useful proxy of atmospheric O 2 levels [5] , [6] , [11] . Under an oxidizing atmosphere, the redox-sensitive elements in continental crust (for example, Os, Re and Mo) are mobilized in the hydrological cycle by oxidative weathering, leading to high concentrations in sediments deposited within anoxic oceans [11] . Under an anoxic atmosphere, in contrast, redox-sensitive elements do not enter the oceans through continental weathering [11] . We propose that records of the abundance of the redox-sensitive element Os and its initial 187 Os/ 188 Os values in sedimentary rocks represent a promising tool for reconstructing variations in atmospheric O 2 during the Great Oxidation Event. Continental sulphides and granites contain high levels of radiogenic 187 Os (currently, 187 Os/ 188 Os~1.4) [12] , [13] . Accordingly, onset of the oxidative delivery of continental Os to the oceans would be recorded as a rise in 187 Os/ 188 Os value in sediments [12] relative to the value dominated by non-radiogenic mantle-derived and extraterrestrial sources of Os ( 187 Os/ 188 Os≈0.11 in the Palaeoproterozoic) [12] . In addition, because the redox potential for the oxidization of Os is higher than that of conventional redox-sensitive elements (Mo and Re), the records of Os abundance in sedimentary rock may allow us to reconstruct the accumulation of high levels of atmospheric O 2 . In fact, studies of the Os isotopic compositions of 2.50-Ga organic-rich shales [11] and of authigenic pyrite in 2.32 Ga shales [14] show no clear evidence of the oxidative weathering of Os, but Mo and Re enrichments are found in the 2.50-Ga organic-rich shale [11] . In the present study, we analysed the abundances of redox-sensitive elements (Os, Re, Mo and U) and Os isotopic compositions in sediments deposited during and after the second Palaeoproterozoic glaciation, to evaluate the role of climate change in the rise of atmospheric O 2 . We focus on shallow-marine sediments, because the signal of the onset of oxidative weathering of Os would first appear in shallow-marine environments [15] , [16] . We found the enhancements of Re, Mo and Os with high initial 187 Os/ 188 Os in the sediments, suggesting that the oxidative delivery of these elements to shallow-marine environments has started in the period of climatic recovery from the second Palaeoproterozoic glaciation. Sampling and the geological setting The Huronian Supergroup is a sequence of early Palaeoproterozoic sediments and minor volcanic rocks. The studied samples were collected from the Bruce and Espanola formations of the 2.45–2.22 Ga Huronian Supergroup [1] , [17] ( Fig. 1 ). Presences of detrital pyrite and uraninite in the lower units of the Huronian Supergroup suggest low O 2 levels in the atmosphere at the time of deposition [1] ; meanwhile, both presence of redbeds and disappearance of mass-independent fractionation in sulphur in the upper units suggest that a significant rise in atmospheric O 2 would have occurred around the second glaciation in the Huronian Supergroup [1] , [8] ( Fig. 1a ). 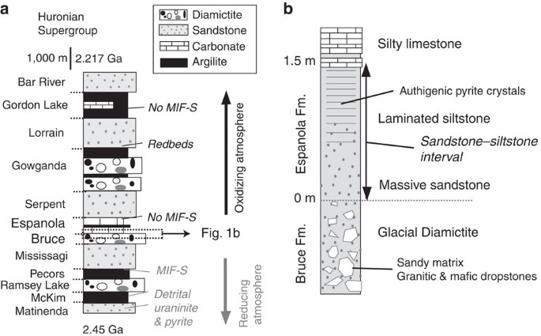Figure 1: Stratigraphy of the Huronian Supergroup. (a) Simplified stratigraphy of the Huronian Supergroup1, showing proxy indicators of redox conditions in the atmosphere1,8. The depositional age of the Huronian Supergroup is constrained to between about 2.45 and 2.217 Ga, based on the dating of dyke swarms in basement rocks and the post-Huronian Nipissing diabase, respectively1,2. Detrital uraninite and pyrite and mass-independent fractionation in sulphur (MIF-S) are found in the lower units1,8; whereas, presence of redbeds and disappearance of MIF-S are observed in the upper units1,8. (b) Stratigraphy of the boundary between the Bruce and Espanola formations. The Bruce Formation contains granitic and mafic dropstones of up to cobble size, in a matrix of grey-green sandstone. The boundary is defined as the uppermost occurrence of dropstones. Figure 1: Stratigraphy of the Huronian Supergroup. ( a ) Simplified stratigraphy of the Huronian Supergroup [1] , showing proxy indicators of redox conditions in the atmosphere [1] , [8] . The depositional age of the Huronian Supergroup is constrained to between about 2.45 and 2.217 Ga, based on the dating of dyke swarms in basement rocks and the post-Huronian Nipissing diabase, respectively [1] , [2] . Detrital uraninite and pyrite and mass-independent fractionation in sulphur (MIF-S) are found in the lower units 1,8 ; whereas, presence of redbeds and disappearance of MIF-S are observed in the upper units 1,8 . ( b ) Stratigraphy of the boundary between the Bruce and Espanola formations. The Bruce Formation contains granitic and mafic dropstones of up to cobble size, in a matrix of grey-green sandstone. The boundary is defined as the uppermost occurrence of dropstones. Full size image The sampling site of the present study is located in the western part of the Huronian Supergroup (called the Elliot Lake area) ( Supplementary Fig. S1 ), where the boundary between the Bruce and Espanola formations is exposed on the east side of Highway 108 (refs 17 , 18 ) (46.248°N, 82.402°W). At the sampling site, a sandstone–siltstone interval (~1.5 m thick) separates diamictites of the underlying Bruce Formation from laminated limestone of the overlying Espanola Formation [18] ( Fig. 1b ). The relatively sudden change from glacial diamictite of the Bruce Formation to carbonate of the Espanola Formation implies a climatic shift from icehouse to greenhouse conditions. The lower part of the sandstone–siltstone interval consists of massive sandstone that changes upward to laminated siltstone, probably reflecting upward deepening associated with a post-glacial marine transgression in a shallow-marine environment [18] . Individual and clustered authigenic sulphide crystals with diameters of ~100 μm or less are observed parallel to laminae in the sandstone–siltstone interval ( Supplementary Fig. S2 ; Supplementary Note 1 ). We analysed isotopic compositions of Os and Re, abundances of Os and other redox–sensitive transition elements, Re, Mo and U in the bulk rock samples (Methods). Total sulphur (TS) and total organic carbon (TOC) contents and carbon isotopic ratio in TOC (δ 13 C org ) in the bulk rock samples are also analysed (Methods). The surfaces of the whole rock samples were cut off and polished with corundum powders to remove potential contaminants. Then, the rocks were cleaned with ultrasonic. The cleaned samples (~2–4 g) were crushed with an agate mortar. For diamictite samples, we removed dropstones and used the sandstone-matrix. The regional settings and rock description are also described in Supplementary Notes 1 and 2 . The results of analyses are summarized in Supplementary Tables S1-S3 . 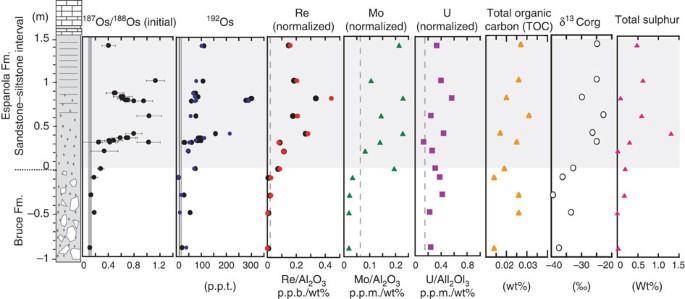Figure 2: Geochemical trends across the Bruce–Espanola boundary. Initial187Os/188Os values, abundances of redox-sensitive elements, TOC content, carbon isotopic values in TOC (δ13Corg), and total sulphur content are shown. Light grey area represents the sandstone–siltstone interval. The average192Os concentrations in upper continental crust12and oceanic basalt20are shown as dark and light lines, respectively, in the plot showing Os concentration. Dashed lines show average Re, Mo and U concentrations normalized by Al2O3in upper continental crust34. Initial187Os/188Os values were obtained based on a depositional age of 2.3±0.2 Ga. The grey line in the plot showing initial187Os/188Os represents the value of mantle-derived components at the time of deposition20. The errors in the initial187Os/188Os values are mainly derived from the errors in depositional age. Black circles in the192Os and Re plots represent the results using inverse aqua regia dissolution media, and red and blue circles represent those using chromium-sulphuric acid. Geochemical trend of the Bruce-Espanola boundary Figure 2 shows variations in the abundances of Os (non-radiogenic 192 Os), Re, Mo and U across the boundary between the Bruce and Espanola formations (herein referred to as the Bruce–Espanola boundary). In the sandstone–siltstone interval, 192 Os abundance is enriched by a factor of 2–20 relative to levels in typical upper continental crust and oceanic basalt. We used chromium-sulphuric acid and inverse aqua regia as dissolution media in Re–Os analyses (Methods and Supplementary Note 3 ). Given that chromium-sulphuric acid dissolves detrital components much less efficiently than does inverse aqua regia, the similarity of the results obtained using the different media ( Fig. 2 ) indicates that the enrichment in Os (and Re) is not related to the detrital component. In addition, the Os concentration in cobbles (which is representative of the average Os concentration of the detrital component) in the diamictites is very low ( 192 Os≈4 p.p.t.) compared with that in the bulk sediments ( 192 Os~10–300 p.p.t.). These results indicate the authigenic enrichment of Os in the sediments. The sandstone–siltstone interval is also marked by high levels of Re and Mo ( Fig. 2 ), which is consistent with the oxidative weathering of redox-sensitive elements and subsequent incorporation in the sediments [19] . Given the correlation between Os abundance and TS content in the sediments ( Fig. 2 ; Supplementary Fig. S3 ), a large component of the Os in the sandstone–siltstone interval is hosted by authigenic sulphide minerals ( Supplementary Note 2 ). These suggest that such minerals are good indicators of the Os isotopic composition of post-glacial bottom water and pore water in sediments. Figure 2: Geochemical trends across the Bruce–Espanola boundary. Initial 187 Os/ 188 Os values, abundances of redox-sensitive elements, TOC content, carbon isotopic values in TOC (δ 13 C org ), and total sulphur content are shown. Light grey area represents the sandstone–siltstone interval. The average 192 Os concentrations in upper continental crust [12] and oceanic basalt [20] are shown as dark and light lines, respectively, in the plot showing Os concentration. Dashed lines show average Re, Mo and U concentrations normalized by Al 2 O 3 in upper continental crust [34] . Initial 187 Os/ 188 Os values were obtained based on a depositional age of 2.3±0.2 Ga. The grey line in the plot showing initial 187 Os/ 188 Os represents the value of mantle-derived components at the time of deposition [20] . The errors in the initial 187 Os/ 188 Os values are mainly derived from the errors in depositional age. Black circles in the 192 Os and Re plots represent the results using inverse aqua regia dissolution media, and red and blue circles represent those using chromium-sulphuric acid. Full size image Based on a depositional age of 2.3±0.2 Ga (an age bound of the Huronian Supergroup), we calculated temporal variations in initial 187 Os/ 188 Os around the Bruce–Espanola boundary ( Fig. 2 ). The initial 187 Os/ 188 Os shows an abrupt increase to ~0.8 at the base of the sandstone–siltstone interval, and varies between 0.4 and 1.1 within the interval; the value within the diamictite is very low, similar to the value of mantle-derived components at ~2.3 Ga (ref. 20 ). The increase in initial 187 Os/ 188 Os in the sandstone–siltstone interval is matched by an increase in Os abundance, strongly indicative of a marked increase in the input of radiogenic Os at the cessation of glaciation. Elevated Os levels in sedimentary rocks might also arise from extraterrestrial [21] , [22] or hydrothermal inputs [23] ; however, these processes typically provide non-radiogenic Os [21] , [23] . The occurrence of much younger alteration would have added Re and radiogenic Os via interaction between oxygenated fluids and organic material in the sediments. However, such interaction would have resulted in a large degree of scatter in the Re–Os isochron plot. Although the scatter in the isochron plot may represent small-scale (<~10 cm; that is, the sample resolution) mobilization of Os and Re by post-depositional alteration, all the data plot within the range expected to develop over a period of 2.3 Ga given initial 187 Os/ 188 Os values that are intermediate between mantle-derived and continental values ( Fig. 3 ; Supplementary Note 4 ). These results do not support the much later addition of radiogenic Os. 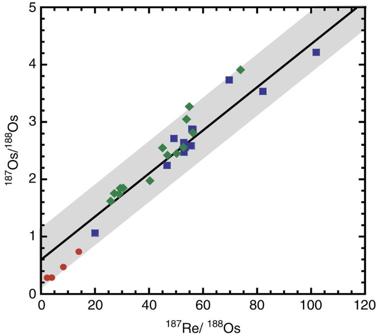Figure 3: Re–Os isochron diagram for the samples. The grey area represents the range of187Re/188Os and187Os/188Os expected to develop over ~2.3 Ga given initial187Os/188Os values of between the mantle-derived (0.11) and continental values (~1.4)12. Colours of the data points represent the positions in the stratigraphy. Red circles represent the samples from the Bruce formation (<0 m from the boundary). Blue squares and green diamonds represent the samples from the lower (0–0.5 m from the boundary) and upper part (0.5–1.5 m from the boudanry) of the sandstone–siltstone interval, respectively. Figure 3: Re–Os isochron diagram for the samples. The grey area represents the range of 187 Re/ 188 Os and 187 Os/ 188 Os expected to develop over ~2.3 Ga given initial 187 Os/ 188 Os values of between the mantle-derived (0.11) and continental values (~1.4) [12] . Colours of the data points represent the positions in the stratigraphy. Red circles represent the samples from the Bruce formation (<0 m from the boundary). Blue squares and green diamonds represent the samples from the lower (0–0.5 m from the boundary) and upper part (0.5–1.5 m from the boudanry) of the sandstone–siltstone interval, respectively. Full size image Given the above observations, we interpret the systematic variations in Os record observed around the Bruce–Espanola boundary to represent evidence for the onset of the oxidative weathering of radiogenic Os on the continents [12] ( Fig. 4 ). We hypothesize that atmospheric O 2 levels increased immediately after the second Palaeoproterozoic glaciation sufficient to mobilize continental Os into the hydrological cycle. Because a large part of the oceans was possibly still anoxic at that time [5] , [24] , the dissolved Os delivered via rivers would have been reduced to immobile Os over a short period, probably before mixing homogeneously in the oceans. In such case, most of the delivered Os would have accumulated within shallow-marine environments ( Fig. 4 ; Supplementary Note 5 ). Within deep-marine environments during the same period, such as the lower Timeball Hill Formation [25] , in contrast, continental Os would have remained depleted because of the short residence time of Os in the anoxic ocean. This would have resulted in the non-radiogenic, hydrothermal Os in the Timeball Hill Formation [14] . 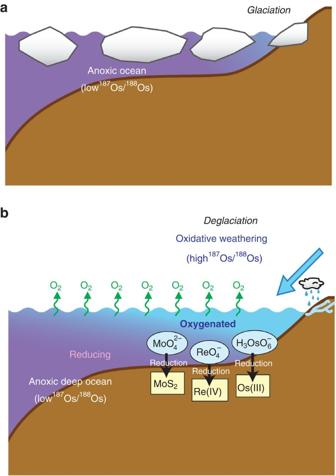Figure 4: Redox conditions of the atmosphere and oceans. (a) During the second Palaeoproterozoic glaciation, the atmospheric O2levels are likely to have been low. It is considered that the shallow-marine environments were also reducing during the glaciation. (b) In the glacial aftermath, the atmospheric O2levels would have become high, sufficient to deliver radiogenic Os to the ocean. The redox-sensitive elements on continents, such as Os, Re and Mo, would have been delivered to the ocean under oxidizing atmospheric conditions and then would have been reduced and deposited in shallow-marine environments, leading to enrichments in the sediments. Figure 4: Redox conditions of the atmosphere and oceans. ( a ) During the second Palaeoproterozoic glaciation, the atmospheric O 2 levels are likely to have been low. It is considered that the shallow-marine environments were also reducing during the glaciation. ( b ) In the glacial aftermath, the atmospheric O 2 levels would have become high, sufficient to deliver radiogenic Os to the ocean. The redox-sensitive elements on continents, such as Os, Re and Mo, would have been delivered to the ocean under oxidizing atmospheric conditions and then would have been reduced and deposited in shallow-marine environments, leading to enrichments in the sediments. Full size image We estimate the O 2 level required for continental Os to enter the oceans, above the level at which Fe 2+ is oxidized to Fe 3+ in soils, as Fe 2+ has a major role as a reductant in converting dissolved Os into immobile Os [26] . Thus, if Fe 2+ is abundant in rivers, little Os would be expected to enter the oceans. Under anoxic atmospheres, soils are a source of Fe 2+ to rivers. To oxidize Fe 2+ to Fe 3+ in soils, atmospheric O 2 should be ≥~10 −4 times the present atmospheric level (PAL) [5] , [6] ; accordingly, O 2 is considered likely to have reached this level. Insoluble U 4+ can be converted to soluble U 6+ under conditions similar that for oxidization of Fe 2+ to Fe 3+ (ref. 27 ) Although a gradual, upward increase in U abundance ( Fig. 2 ) might reflect an increase in soluble U 6+ concentration, low levels of U enrichment relative to those of Re, Mo, and Os imply that atmospheric O 2 would not have substantially exceeded ~10 −4 PAL. Figure 2 also shows that the observed high 187 Os/ 188 Os values seem to decrease in the upper part of this section, whereas those of Mo and Re do not. This also implies that the atmospheric O 2 had been fluctuated around ~10 −4 PAL where Mo and Re is sufficiently delivered to the oceans but Os is not. Previous studies have proposed a possible link between glaciations and the rise in O 2 (refs 2 , 3 , 8 , 9 , 10 ). For example, a global warming in a glacial aftermath may have provided nutrients to the ocean via chemical weathering, leading to a cyanobacterial bloom [8] , [9] , [17] . In fact, the recovery of carbon isotopic values in TOC to ~25‰ preceding Os enrichment ( Fig. 2 ) implies that primary production by photosynthesis has become predominant in the glacial aftermath ( Supplementary Note 6 ). In addition, melting at the glacier base would release H 2 O 2 , which interacts with seawater to form O 2 (ref. 9 ). Our observations support the hypothesis that climatic recovery acted to accelerate atmospheric oxidization [3] , [8] , [9] , [10] . Alternatively, if the rise in O 2 occurred before the second Palaeoproterozoic glaciation, because of increased subaerial volcanism [28] , another explanation is required for the low abundances of redox-sensitive elements and low initial 187 Os/ 188 Os in the Bruce Formation. The Snowball Earth hypothesis [3] , [29] predicts a shutdown of the hydrological cycle, thereby severely restricting the input of redox-sensitive elements into the oceans. To assess the possibility of a Snowball Earth at the time of the glaciation recorded by the Bruce Formation, further palaeomagnetic studies are required. If that is confirmed, it would mean that the Bruce Snowball glaciation preceded the Makganyene Snowball glaciation [2] , [3] in the Palaeoproterozoic, and that Snowball Earth events might have occurred as pairs at both the beginning and end of Proterozoic in Earth's history. Re-Os analysis Sample weights for Re-Os analysis are ~1.0–2.0 g for diamictite and ~0.3 g for the sandstone–siltstone interval. The analytical procedure for the Os and Re concentrations and Os isotopes of this study is based on isotope dilution combined with Carius tube digestion, carbon tetrachloride and solvent extractions, microdistillation, and column separations (for example, refs 20 , 30 ). For each analysis, powdered whole rock samples, mixed with a known amount of 185 Re and 190 Os spike solutions, were dissolved and equilibrated with dissolution medium using the Carius tube method. We used two types of dissolution medium for the Re-Os analysis; chromium-sulphuric acid (5 ml) and inverse aqua regia (10 ml). The chromium-sulphuric acid had to be purified for Re and Os before use. The purification method given by ref. 31 was followed in the present study. After heating sealed Carius tubes at 230 °C for at least 24 h, Os was extracted by carbon tetrachloride and subsequently back-extracted into 9 N HBr. Micro-distillation further purified the extracted Os. Rhenium was separated from the aqueous phase using Muromac's AG 1-X8 anion exchange resin [30] , [32] . The Os and Re isotopic measurements were performed with a ThermoFinnigan TRITON (NTIMS) at JAMSTEC [30] , [32] . The Os was loaded on a high-purity Pt filament that had been baked in air to high temperatures for 3 min before loading. The samples were covered with 10 μg Ba using a 10,000 p.p.m. Ba(NO 3 ) 2 solution. The instrumental mass fractionation of Os was corrected by normalizing the measured 192 Os/ 188 Os ratio to 3.08271 (ref. 30 ). Rhenium isotope ratios were measured with a total evaporation technique [32] . The total blank levels for Re and Os are shown in the note of Supplementary Tables S1 and S2 . The reproducibility of replicate analyses was examined using molybdenite (high Os concentrations) and andesite (low Os concentrations) by ref. 30 . The Re-Os model ages determined for the standard molybdenite samples have an excellent reproducibility of ±0.34% ( n =3, 2 σ) [30] . The Re-Os age for the standard molybdenite samples (221.1±0.8 Ma) is also in excellent agreement with the Re-Os ages of 221.5±0.3 and 221.3±0.2 Ma obtained previously [30] . The 187 Os/ 188 Os ratios and Re and Os concentrations of the five standard andesite samples are 0.2092±0.0078 (2 σ) and 46.7±1.6 and 11.4±1.5 p.p.t., respectively [30] . The reproducibility of the standard andesite samples is also high enough for Re-Os analyses of low-Os samples. More detailed data about the reproducibility are shown in ref. 30 . Major and trace elements Bulk chemical and mineralogical compositions of the rock samples were analysed with standard X-ray fluorescence technologies (AXIOS, PANalytical) and an X-ray Diffractometer (X'PERT-PRO, PANalytical), respectively, at University of Tokyo. For the measurements of Mo and U abundance, we used ~100 mg of the rock powder. The powder samples were digested with HNO 3 , HClO 4 and HF. After evaporation of acids to near dryness, the residues were dissolved in a HNO 3 (2%) and HF (0.1%) solution. The Mo and U abundances in the solutions were measured with an inductive-coupled plasma mass spectrometer (7500ce; Agilent) at JAMSTEC. Sulphur analysis TS analysis for the powder samples was conducted with a helium-gas continuous-flow isotope-ratio mass spectrometer (Isoprime-EA (Isoprime)) at University of Tsukuba. Sample weights for the TS analyses are ~3 mg. TS contents of the samples represent the mean values of four repeated measurements of the powder samples. Errors for the TS contents are obtained from one standard deviation of the repeated measurements. Carbon analysis For TOC and δ 13 C org analyses, the powder samples were treated with 4 M hydrochloric acid for 2 days. Then, they were washed with distilled water several times to remove calcium salt and dried in an oven. Measurements for TOC contents and their carbon isotopic compositions were performed by an on-line system of Finnigan Delta Plus XP isotope-ratio mass spectrometry at JAMSTEC [33] , [35] . Total organic carbon content in the samples was determined by calibrated ion currents of m/z 44, 45, and 46 in isotope ratio mass spectrometry. Carbon isotopic compositions were expressed as conventional δ notation against V-PDB standard; δ 13 C=( 13 R sample / 13 R standard −1)×1,000, where 13 R is 13 C/ 12 C ratio. How to cite this article: Sekine, Y. et al . Osmium evidence for synchronicity between a rise in atmospheric oxygen and Palaeoproterozoic deglaciation. Nat. Commun. 2:502 doi: 10.1038/ncomms1507 (2011).